MYPT1 regulates contractility and microtubule acetylation to modulate integrin adhesions and matrix assembly Although much is known about how individual cytoskeletal systems contribute to physiological processes such as cell migration and branching morphogenesis, little is known about how these different systems actively coordinate their functions after polymerization. Here we show that both fibroblasts and developing glands reciprocally coordinate levels of cellular contractility and microtubule acetylation. We find that this balance is achieved by interaction of the myosin phosphatase target subunit of myosin phosphatase with either myosin light chain or HDAC6, a microtubule deacetylase. This balance of contractility and microtubule acetylation controls progression of adhesion maturation by regulating surface density of α 5 β 1 integrin and fibronectin. Thus, we propose that a homeostatic balance between contractility and microtubule acetylation is mediated by myosin phosphatase via controlled activation and deactivation of myosin II and HDAC6. This regulates the surface density of α 5 β 1 integrin to modulate fibronectin matrix assembly and governs rates of cell migration and branching morphogenesis. Efficient cell migration is achieved only when adhesion to the substratum is executed optimally; too strong or too weak adhesion decreases the efficiency of migration [1] , [2] , [3] . In classical 2D cell migration, integrins, a major class of adhesion receptors that span the plasma membrane [4] , mediate attachment to the substrate [1] , [5] , [6] . Integrin-mediated adhesions form at the leading edge and disassemble at the rear of the cell. By convention, these adhesions are categorized into subclasses defined as nascent, focal and fibrillar adhesions based on their composition, size and localization. Assembly, maturation and disassembly of these adhesions are dictated by ligand and receptor concentration, affinity and avidity of ligand–receptor interactions and integrin recruitment of cytoskeletal components [1] , [2] , [3] . To achieve an optimum migration rate, adhesion assembly must be strategically coupled to adhesion maturation and disassembly. The fate of newly formed adhesions is to mature or to disassemble. A number of parameters affect adhesion maturation, but cellular contractility, which is mediated by actomyosin contraction, plays a key role. The strength of actomyosin contraction is controlled by the cyclical activity of the myosin heavy chain power stroke on actin fibres, which in turn is largely regulated by the phosphorylation and dephosphorylation of regulatory myosin light chain (rMLC) at Ser-19 and Thr-18 (ref. 7 ). Progression of adhesion maturation requires actin and myosin wherein nascent adhesions mature into focal adhesions, which then develop into fibrillar adhesions [8] , [9] , [10] . Fibrillar adhesions then assist fibronectin (FN) fibrillogenesis and matrix assembly [11] , [12] . Thus, promoting the formation of one type of adhesion may perturb the normal progression of adhesion maturation and adhesion disassembly. The other outcome for an adhesion is disassembly, which promotes detachment of cells from the substratum. Although the precise mechanism is not yet elucidated, adhesions disassemble by dissolution of adhesion components by endocytosis of integrins [13] and/or degradation of adhesion components via calpain-mediated proteolysis [14] , both of which require microtubules. In fact, plus-end microtubule targeting to focal adhesions is important for adhesions to dissipate [15] , [16] , [17] . Alternatively, cells can detach from the substratum without disassembling adhesions by simply increasing contractility and mechanically pulling or ‘ripping’ the cell away from its attachments [2] . Thus, cells appear to use contractility and microtubules to modulate their attachment and detachment from substrata. These seemingly opposing actions of actomyosin-mediated cellular contractility and microtubules suggest that the two cytoskeletal systems must coordinate their functions to promote effective migration; too much or too little adhesion impedes locomotion. We report here a novel reciprocal interplay between contractility and microtubule acetylation in cultured fibroblasts and a branching organ. This interplay is achieved through mutually exclusive interaction of the myosin phosphatase target subunit (MYPT1) of myosin phosphatase with either a regulatory myosin light chain (rMLC) or a microtubule deacetylase (HDAC6) to regulate the surface density of α 5 β 1 integrin and FN to modulate matrix assembly. We find that coordination between cellular contractility and microtubule acetylation governs the rate of cell migration and branching morphogenesis. Linkage of contractility and microtubule acetylation A previous observation that the level of microtubule acetylation is elevated after inhibition or ablation of myosin IIA [18] led us to hypothesize that cells may coordinate levels of cellular contractility and microtubule acetylation. As the first test of this hypothesis, we searched for evidence of regulatory effects on actomyosin contractility by evaluating levels of myosin light chain phosphorylation. We inhibited actomyosin contractility by treating human foreskin fibroblasts (HFFs) with either blebbistatin (Bleb), a myosin II ATPase inhibitor, or ML-7, a myosin light chain kinase inhibitor [19] , and found that either treatment increased the level of microtubule acetylation ( Fig. 1a,b ). In contrast, calyculin A (CalA), which increases contractility by inhibiting myosin phosphatase [20] , suppressed microtubule acetylation. Conversely, to investigate whether altering the level of microtubule acetylation affects cellular contractility, we measured changes in the phosphorylation of regulatory myosin light chain (rMLC) at Ser-19 as an evidence for a regulatory effect on contractility. Treatment with trichostatin A (TSA), an inhibitor of HDACs, decreased the level of phosphorylated rMLC (pMLC; Fig. 1b,c ). Blebbistatin treatment increased pMLC level in our system, consistent with previous findings with this drug [21] . Furthermore, levels of pMLC decreased with increasing microtubule acetylation due to TSA treatment, and acetylation decreased with increasing calyculin A, respectively, consistent with a biologically relevant linkage of these post-translational modifications after drug treatment ( Supplementary Fig. 1a,b ). 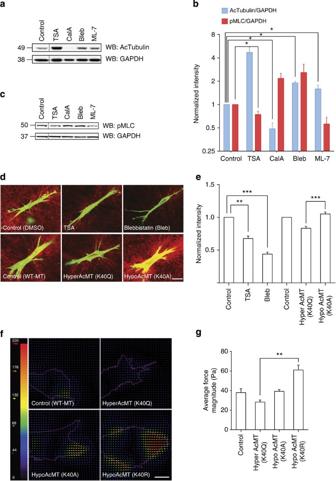Figure 1: Fibroblasts reciprocally balance cellular contractility and microtubule acetylation. (a,c) Representative western blots of cell lysates of HFFs treated with the indicated reagents. (b) Quantification ofaandc. Relative levels of acetylated microtubules or phosphorylated MLC, each normalized against GAPDH (n>3 experiments per condition). (d) Representative confocal images of HFFs cultured in 3D collagen then treated as indicated, or HFFs transiently expressing GFP-tagged wild-type tubulin (control, WT-MT), GFP-tagged acetyl-mimetic mutant of tubulin (α-tubulin K40Q; HyperAcMT) or GFP-tagged acetyl-null tubulin mutant (α-tubulin K40A; HypoAcMT). F-actin and collagen fibres were visualized by rhodamine-phalloidin (green) or confocal reflection microscopy (red), respectively. All images were acquired using identical instrument settings. (e) Quantification of reflection intensity by collagen fibres ind, expressed as intensity compared with the control. Ten cells were counted for each drug treatment study, and more than 70 cells were counted for each experiment (n>3). (f) Examples of force traction maps of HFFs stably expressing different tubulin mutants. HypoAcMT (K40R) represents another type of acetyl-null tubulin mutation that allows maintenance of the overall shape and positive charge of the K-40 residue. The colours and numbers indicate local traction force in Pascals; cell outlines are indicated by purple lines. (g) Quantification of average traction force magnitude per cell in Pascals (n>8). Data are shown as mean±s.e.m. *P<0.05; **P<0.01; ***P<0.001. Student’st-test was used forb, and two-way analysis of variance (ANOVA) followed by Tukeypost testwas used foreandg. (d) Scale bar, 50 μm; (f) scale bar, 20 μm. Figure 1: Fibroblasts reciprocally balance cellular contractility and microtubule acetylation. ( a , c ) Representative western blots of cell lysates of HFFs treated with the indicated reagents. ( b ) Quantification of a and c . Relative levels of acetylated microtubules or phosphorylated MLC, each normalized against GAPDH ( n >3 experiments per condition). ( d ) Representative confocal images of HFFs cultured in 3D collagen then treated as indicated, or HFFs transiently expressing GFP-tagged wild-type tubulin (control, WT-MT), GFP-tagged acetyl-mimetic mutant of tubulin (α-tubulin K40Q; HyperAcMT) or GFP-tagged acetyl-null tubulin mutant (α-tubulin K40A; HypoAcMT). F-actin and collagen fibres were visualized by rhodamine-phalloidin (green) or confocal reflection microscopy (red), respectively. All images were acquired using identical instrument settings. ( e ) Quantification of reflection intensity by collagen fibres in d , expressed as intensity compared with the control. Ten cells were counted for each drug treatment study, and more than 70 cells were counted for each experiment ( n >3). ( f ) Examples of force traction maps of HFFs stably expressing different tubulin mutants. HypoAcMT (K40R) represents another type of acetyl-null tubulin mutation that allows maintenance of the overall shape and positive charge of the K-40 residue. The colours and numbers indicate local traction force in Pascals; cell outlines are indicated by purple lines. ( g ) Quantification of average traction force magnitude per cell in Pascals ( n >8). Data are shown as mean±s.e.m. * P <0.05; ** P <0.01; *** P <0.001. Student’s t -test was used for b , and two-way analysis of variance (ANOVA) followed by Tukey post test was used for e and g . ( d ) Scale bar, 50 μm; ( f ) scale bar, 20 μm. Full size image To confirm that microtubule acetylation changes cellular contractility, we used two well-established biophysical methods: collagen gel contraction and traction force assays. First, traditional 3D collagen gel contraction assays have been used to indicate cellular contraction because contracting cells rearrange and compact collagen fibres [22] , [23] . However, this assay requires large numbers of cells. Since the denser collagen fibres scatter more light such that greater reflectance is observed from more-contractile cells in collagen [24] , we analysed locally increased density of a collagen gel matrix as a measure of cellular contractility. As expected, loss of contractility after blebbistatin treatment reduced collagen density compared with the control ( Fig. 1d,e ). Notably, TSA treatment also reduced the density of collagen at the cell surface, which serves as an evidence for a decrease in cellular contractility. Since TSA inhibits other HDACs that are not involved in microtubule deacetylation, it was essential to establish directly whether acetylation of microtubules reduced cellular contraction. Thus, we generated mutations at Lys-40 of α-tubulin to mimic acetylated or non-acetylated states [25] , [26] and evaluated cellular contractility. Expression of the acetyl-mimetic mutant of tubulin (α-tubulin K40Q; HyperAcMT) resulted in reduced contracted collagen accumulation, whereas expression of the acetyl-null tubulin mutant (α-tubulin K40A; HypoAcMT) increased local collagen accumulation ( Fig. 1d,e ), recapitulating the results of drug treatments. These changes in cellular contractility after expression of different tubulin mutants were verified by a second method that measures tensional force generated by cells on a reporter substrate. We found that cells expressing HyperAcMT displayed a lower magnitude of average force compared with elevated traction force by cells expressing the K40R HypoAcMT mutant ( Fig. 1f,g ). Together, these three independent assays suggest reciprocal and bidirectional cross-talk between microtubule acetylation and cellular contractility. To further validate these findings, we exploited the fact that cells modulate cellular contractility to match their surroundings: greater contractility is measured in cells plated on rigid surfaces compared with those on softer surfaces [27] . A decrease in acetylated microtubules was observed when HFFs were seeded on a rigid surface (1 GPa) compared with those that were seeded on a softer surface (28 kPa; Supplementary Fig. 1c–e ). Conversely, the rigid surface induced higher phosphorylation of MLC compared with the softer surface ( Supplementary Fig. 1f ). More importantly, cells stably expressing HyperAcMT decreased pMLC levels ( Supplementary Fig. 1g ). Altogether, these data suggest that HFFs reciprocally balance the levels of cellular contractility and microtubule acetylation. MYPT1 modulates contractility and microtubule deacetylation Dephosphorylation of rMLC is regulated by myosin phosphatase, a protein complex composed of a myosin phosphatase target subunit (MYPT1), a catalytic domain (PP1δ) and a non-catalytic domain [28] . Interestingly, activity of HDAC6 is also regulated by phosphorylation, possibly at Ser-22 (refs 29 , 30 ). HDAC6 binds directly to protein phosphatase 1 (PP1) in vitro [29] , yet phosphatases normally require a substrate-binding subunit to specify their substrates in vivo [31] . Consequently, we theorized that myosin phosphatase may also dephosphorylate HDAC6 and modulate its activity by first interacting with MYPT1. Indeed, MYPT1 coimmunoprecipitated with HDAC6 ( Fig. 2a ), and recombinant HDAC6 protein directly interacted with immobilized GST-tagged MYPT1 ( Fig. 2b ). Treatment with TSA inhibited HDAC6-MYPT1 complex formation, whereas sodium butyrate (NaB, another general HDAC inhibitor that does not inhibit HDAC6), did not ( Fig. 2a ). This inhibition of complex formation after drug treatment was also observed in a reciprocal immunoprecipitation analysis in which HDAC6 coimmunoprecipitated with MYPT1 ( Supplementary Fig. 2a ). Importantly, blebbistatin treatment also reduced HDAC6–MYPT1 complex formation ( Supplementary Fig. 2a ). Conversely, treatment with calyculin A (CalA) increased the HDAC6–MYPT1 complex formation ( Supplementary Fig. 2b ). This decrease or increase in the HDAC6-MYPT1 complex was accompanied by a concomitant increase or decrease, respectively, in MLC–MYPT1 complex formation ( Fig. 2c and Supplementary Fig. 2c ). Furthermore, addition of purified recombinant HDAC6 to HFF lysates decreased the MLC–MYPT1 complex, indicating a competitive interaction between MLC and HDAC6 with MYPT1 ( Fig. 2d ). 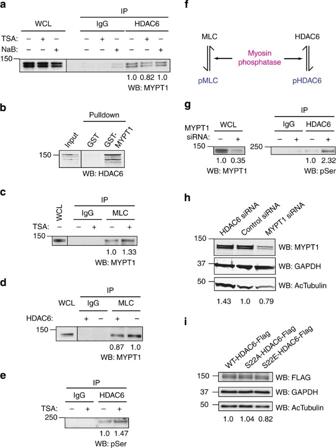Figure 2: MYPT1 functions as a switch to regulate contractility and microtubule acetylation. (a) Representative western blot probed with an anti-MYPT1 antibody after immunoprecipitating HDAC6 after the indicated treatments. Two percent of input (whole-cell lysate, WCL) and 50% of the immunoprecipitates were loaded. Intensities of immunoprecipitated bands were 0.82±0.07 (TSA) and 1.00±0.09 (NaB) compared with the control (1.0;n=3). (b) Representative western blot of GST pull-down of soluble recombinant HDAC6 using recombinant MYPT1 immobilized on glutathione-agarose beads at an equal molar ratio. Five percent of the input and 50% of the pull-downs were loaded and probed with the indicated antibody. (c) Western blot after immunoprecipitating MLC with TSA treatment and probed with an anti-MYPT1 antibody. Two percent of input (whole-cell lysate, WCL) and 50% of the immunoprecipitates were loaded. (d) Representative western blot after immunoprecipitating MLC in the presence of purified recombinant HDAC6. Five percent of input and 100% of immunoprecipitates were loaded and probed with an anti-MYPT1 antibody. Intensity of immunoprecipitated band was 0.87±0.05 compared with the control (1.0;n=4). (e) Representative western blot after immunoprecipitating HDAC6 with TSA treatment and probed with an anti-pSer antibody. Fifty percent of the immunoprecipitates were loaded. Intensity of immunoprecipitated band was 1.47±0.20 compared with the control (1.0;n=4). (f) Schematic summary of findings ina–e. (g) Western blot of HDAC6 immunoprecipitates from HFFs transfected with scrambled siRNA (control siRNA) or siRNA silencing MYPT1 and then probed with the indicated antibodies. Two percent of the input (WCL) and 100% of the immunoprecipitates were loaded. Intensity of MYPT1 band after transfection was 0.35±0.04 compared with the control (1.0;n=7), and immunoprecipitated band was 2.32±0.27 compared with the control (1.0;n=4). (h) Western blot of whole-cell lysates from cells transfected with scrambled siRNA (control siRNA), siRNA silencing HDAC6 or siRNA silencing MYPT1. Each lysate was probed with the indicated antibodies. Intensity of each band probed with an anti-acetylated tubulin antibody normalized against GAPDH was 1.43±0.21 (HDAC6 siRNA), 0.79±0.11 (MYPT1 siRNA) compared with the control (1.0;n=3). (i) Western blot of whole-cell lysates from cells overexpressing HDAC6 mutated at Ser-22, as indicated in each lane, and probed with the indicated antibodies. Intensity of each bands probed with an anti-acetylated tubulin antibody normalized against GAPDH were 1.04±0.09 (S22A-HDAC6-Flag), 0.82±0.12 (S22E-HDAC6-Flag) compared with the control (1.0;n>6). Data are mean±s.e.m. Figure 2: MYPT1 functions as a switch to regulate contractility and microtubule acetylation. ( a ) Representative western blot probed with an anti-MYPT1 antibody after immunoprecipitating HDAC6 after the indicated treatments. Two percent of input (whole-cell lysate, WCL) and 50% of the immunoprecipitates were loaded. Intensities of immunoprecipitated bands were 0.82±0.07 (TSA) and 1.00±0.09 (NaB) compared with the control (1.0; n =3). ( b ) Representative western blot of GST pull-down of soluble recombinant HDAC6 using recombinant MYPT1 immobilized on glutathione-agarose beads at an equal molar ratio. Five percent of the input and 50% of the pull-downs were loaded and probed with the indicated antibody. ( c ) Western blot after immunoprecipitating MLC with TSA treatment and probed with an anti-MYPT1 antibody. Two percent of input (whole-cell lysate, WCL) and 50% of the immunoprecipitates were loaded. ( d ) Representative western blot after immunoprecipitating MLC in the presence of purified recombinant HDAC6. Five percent of input and 100% of immunoprecipitates were loaded and probed with an anti-MYPT1 antibody. Intensity of immunoprecipitated band was 0.87±0.05 compared with the control (1.0; n =4). ( e ) Representative western blot after immunoprecipitating HDAC6 with TSA treatment and probed with an anti-pSer antibody. Fifty percent of the immunoprecipitates were loaded. Intensity of immunoprecipitated band was 1.47±0.20 compared with the control (1.0; n =4). ( f ) Schematic summary of findings in a – e . ( g ) Western blot of HDAC6 immunoprecipitates from HFFs transfected with scrambled siRNA (control siRNA) or siRNA silencing MYPT1 and then probed with the indicated antibodies. Two percent of the input (WCL) and 100% of the immunoprecipitates were loaded. Intensity of MYPT1 band after transfection was 0.35±0.04 compared with the control (1.0; n =7), and immunoprecipitated band was 2.32±0.27 compared with the control (1.0; n =4). ( h ) Western blot of whole-cell lysates from cells transfected with scrambled siRNA (control siRNA), siRNA silencing HDAC6 or siRNA silencing MYPT1. Each lysate was probed with the indicated antibodies. Intensity of each band probed with an anti-acetylated tubulin antibody normalized against GAPDH was 1.43±0.21 (HDAC6 siRNA), 0.79±0.11 (MYPT1 siRNA) compared with the control (1.0; n =3). ( i ) Western blot of whole-cell lysates from cells overexpressing HDAC6 mutated at Ser-22, as indicated in each lane, and probed with the indicated antibodies. Intensity of each bands probed with an anti-acetylated tubulin antibody normalized against GAPDH were 1.04±0.09 (S22A-HDAC6-Flag), 0.82±0.12 (S22E-HDAC6-Flag) compared with the control (1.0; n >6). Data are mean±s.e.m. Full size image We also observed a corroborative increase in phosphorylated HDAC6 at Ser-22 and/or Ser-1,035 accompanying the decrease in the HDAC6–MYPT1 complex ( Fig. 2e ), suggesting that the interaction of HDAC6 with MYPT1 alters the phosphorylation state of HDAC6. Moreover, calyculin A treatment prevented dephosphorylation of HDAC6, even though the amount of HDAC6–MYPT1 complex increased ( Supplementary Fig. 2d ). These results predict that a lack of MYPT1 protein should increase phosphorylation of HDAC6, which should then decrease the level of acetylated microtubules ( Fig. 2f ). Indeed, knockdown of MYPT1 with MYPT1 siRNA both increased phosphorylated HDAC6 ( Fig. 2g ) and decreased the level of acetylated microtubules ( Fig. 2h ). To investigate whether phosphorylation at Ser-22 on HDAC6 enhanced the enzyme activity of HDAC6, we generated a phospho-mimetic mutant (S22E) of HDAC6 and assayed its ability to decrease acetylation of microtubules in fibroblasts. Expression of this mutant decreased the level of acetylated microtubules, that is, S22E mutation augmented enzymatic activity of HDAC6 ( Fig. 2i ). Conversely, expression of the phospho-null mutant (S22A) of HDAC6 slightly increased the level of acetylated microtubules, consistent with loss of HDAC6 enzyme activity without Ser-22 phosphorylation. Altogether, these data demonstrate that MYPT1 and HDAC6 interact directly to regulate the enzymatic activity of HDAC6 by controlling dephosphorylation at Ser-22. Migration requires balanced contractility and MT acetylation Inhibition or ablation of HDAC6 impedes cell migration, but whether this decrease is due to HDAC6 protein itself or microtubule acetylation is not known [32] , [33] . Thus, to decipher the role of microtubule acetylation in cell migration, we expressed α-tubulin K40Q (HyperAcMT) or α-tubulin K40A (HypoAcMT) in HFFs and tested the ability of expressing cells to migrate. Cells expressing HyperAcMT migrated at only half the velocity of cells expressing HypoAcMT ( Fig. 3a ). Importantly, expression of these different mutants of tubulins comprised only a subfraction of total tubulin and had no effects on overall microtubule dynamics or organization ( Supplementary Fig. 3 and Supplementary Table 1 ). Thus, microtubule acetylation can inhibit cell migration without affecting overall microtubule dynamics. 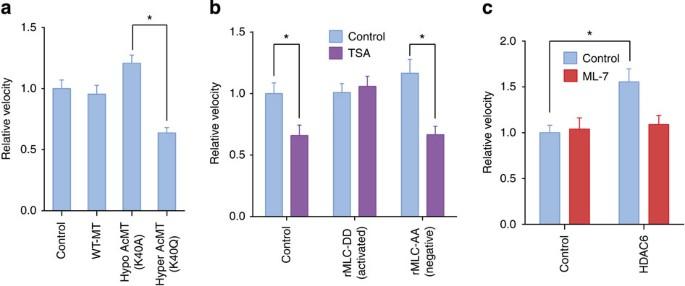Figure 3: Inhibition of migration due to increased acetylation of microtubules can be rescued by counterbalancing with increased contractility. (a) Relative migration velocity of HFFs stably expressing GFP (control) or different tubulins as indicated. Velocities were normalized to the control. A minimum of 50 time points were used per measurement from >30 cells (n>3). (b) Relative migration velocity of TSA-treated HFFs (5 μM TSA) expressing GFP (control), GFP-tagged phospho-mimetic MLC (rMLC-DD; activated) or GFP-tagged phospho-null MLC (rMLC-AA; negative). Velocities were normalized to the control. A minimum of 40 time points were used per measurement from >20 cells (n=3). (c) Relative migration velocity of HFFs expressing Flag-tagged HDAC6 treated with 20 μM ML-7. Each velocity was normalized to the control. A minimum of 30 time points were used per measurement from >45 cells (n=3). Data are mean±s.e.m.*P<0.05. Two-way analysis of variance (ANOVA) followed by Tukeypost testwas used fora, and Student’st-test was used forbandc. Figure 3: Inhibition of migration due to increased acetylation of microtubules can be rescued by counterbalancing with increased contractility. ( a ) Relative migration velocity of HFFs stably expressing GFP (control) or different tubulins as indicated. Velocities were normalized to the control. A minimum of 50 time points were used per measurement from >30 cells ( n >3). ( b ) Relative migration velocity of TSA-treated HFFs (5 μM TSA) expressing GFP (control), GFP-tagged phospho-mimetic MLC (rMLC-DD; activated) or GFP-tagged phospho-null MLC (rMLC-AA; negative). Velocities were normalized to the control. A minimum of 40 time points were used per measurement from >20 cells ( n =3). ( c ) Relative migration velocity of HFFs expressing Flag-tagged HDAC6 treated with 20 μM ML-7. Each velocity was normalized to the control. A minimum of 30 time points were used per measurement from >45 cells ( n =3). Data are mean±s.e.m. * P <0.05. Two-way analysis of variance (ANOVA) followed by Tukey post test was used for a , and Student’s t -test was used for b and c . Full size image Our data indicate that increased microtubule acetylation reduces cellular contractility ( Fig. 1 ). Since high contractility can pull cells away from tight cell adhesions at the rear of migrating cells [2] , we asked whether the decrease in migration velocity upon microtubule acetylation could be rescued by increasing actomyosin contraction. This would re-establish the proposed cellular balance between contractility and microtubule acetylation, but with higher levels of each. To test our hypothesis, we transfected cells with activated or inactive myosin light chain. We compared migration velocities of fibroblasts expressing GFP (control), GFP-tagged rMLC-T18D/S19D (rMLC-DD; activated) or GFP-tagged rMLC-T18A/S19A (rMLC-AA; negative) with TSA treatment. Expression of rMLC-DD protected cells from the TSA-induced decrease in migration velocity, whereas expression of rMLC-AA could not counter the TSA-induced migration defect ( Fig. 3b ). Conversely, overexpression of the tubulin deacetylase HDAC6 increased migration rate, and this enhancement was restored to normal after treatment with ML-7 ( Fig. 3c ). Together, these data suggest that a homeostatic balance of contractility and microtubule acetylation is needed to achieve a normal rate of cell migration, that disruption of the balance affects migration velocity, and that the defects in migration velocity can be rescued by counterbalancing changes in the other cytoskeletal system. Adhesion disassembly is inhibited by microtubule acetylation Fibroblast migration is controlled by adhesion maturation and turnover, which in turn is regulated by actomyosin contraction and microtubules [1] , [5] , [34] . Hence, we investigated whether the balance between contractility and microtubule acetylation affects adhesions. First, we examined cell-matrix adhesions when the balance was perturbed by expressing HyperAcMT or K40A HypoAcMT ( Fig. 1 ). Expression of different tubulins did not grossly disrupt adhesions containing α v β 3 integrin and phosphotyrosine ( Supplementary Fig. 4a,b ), which are used to identify focal adhesions [12] . However, expression of HyperAcMT significantly increased the number of long paxillin-containing adhesions ( Fig. 4a ). When the axial ratio of paxillin-containing adhesions was quantified, expression of HyperAcMT resulted in 19.7±3.9% (s.e.m.) elongated adhesions (axial ratio >4) [35] compared with 10.8±1.8% (s.e.m.) in cells expressing K40A HypoAcMT ( Fig. 4b ). This result implies that expression of HyperAcMT promotes the formation of elongated fibrillar adhesions. 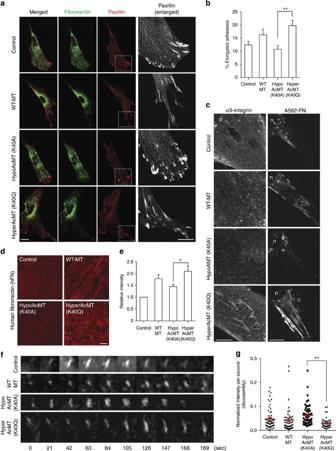Figure 4: Acetylation of microtubules decreases adhesion disassembly and promotes adhesion maturation. (a) Representative confocal images of HFFs expressing GFP (control) or different tubulins as indicated immunostained for FN (green) and paxillin (red). Front of cell (hatched box) enlarged in the right panels. (b) Quantification of elongated adhesions inafrom a minimum of 25 cells (n=3). (c) Representative confocal images of HFFs expressing the indicated tubulin mutants and immunostained with anti-α5integrin (left panels) or incubated overnight with Alexa Fluor 562-labelled FN (right panels;n=nucleus). (d) Maximally projected confocal images of matrices derived from cells expressing the indicated tubulin mutants and immunostained for human FN (antibody 3B8). (e) Human FN from matrices described indquantified by western blot as relative intensity (n=4). (f) Representative confocal spinning disc images of HFFs expressing different tubulins as indicated with mApple-paxillin; see alsoSupplementary Movie 1. (g) Scatter plot of disassembly rate of adhesions fromf. Data are mean (red bars) ±s.e.m. *P<0.05 and **P<0.01. Two-way analysis of variance (ANOVA) followed by Tukeypost testwas used forb,eandg. Scale bar, 20 μm (a; left panels); scale bar, 10 μm (a; right panels andc); scale bar, 100 μm (d); scale bar, 5 μm (f). Figure 4: Acetylation of microtubules decreases adhesion disassembly and promotes adhesion maturation. ( a ) Representative confocal images of HFFs expressing GFP (control) or different tubulins as indicated immunostained for FN (green) and paxillin (red). Front of cell (hatched box) enlarged in the right panels. ( b ) Quantification of elongated adhesions in a from a minimum of 25 cells ( n =3). ( c ) Representative confocal images of HFFs expressing the indicated tubulin mutants and immunostained with anti-α 5 integrin (left panels) or incubated overnight with Alexa Fluor 562-labelled FN (right panels; n =nucleus). ( d ) Maximally projected confocal images of matrices derived from cells expressing the indicated tubulin mutants and immunostained for human FN (antibody 3B8). ( e ) Human FN from matrices described in d quantified by western blot as relative intensity ( n =4). ( f ) Representative confocal spinning disc images of HFFs expressing different tubulins as indicated with mApple-paxillin; see also Supplementary Movie 1 . ( g ) Scatter plot of disassembly rate of adhesions from f . Data are mean (red bars) ±s.e.m. * P <0.05 and ** P <0.01. Two-way analysis of variance (ANOVA) followed by Tukey post test was used for b , e and g . Scale bar, 20 μm ( a ; left panels); scale bar, 10 μm ( a ; right panels and c ); scale bar, 100 μm ( d ); scale bar, 5 μm ( f ). Full size image To determine whether these increased elongated paxillin-containing adhesions were fibrillar adhesions, we immunostained for α 5 β 1 and visualized incorporation of FN, which are characteristics of fibrillar adhesions [11] , [12] . HFFs expressing HyperAcMT showed more α 5 β 1 integrin-positive adhesions and FN fibrillogenesis ( Fig. 4c ). Also, more FN fibrils could be detected on cells plated on a soft surface ( Supplementary Fig. 1e ). These data suggest that acetylation of microtubules, which decreases contractility ( Fig. 1 ), promotes adhesion maturation into fibrillar adhesions. Fibrillar adhesions assist in FN fibrillogenesis and matrix assembly [11] , [12] . Therefore, we evaluated overall FN fibrillogenesis by examining cell-derived matrices from HFFs expressing different tubulin mutants [36] . These cell-derived matrices are mainly composed of FN that is secreted by cells and do not contain cells or functional cytoskeletal proteins [36] . HFFs expressing HyperAcMT had more total FN than the cells expressing K40A HypoAcMT as indicated by fluorescence intensities from micrographs ( Fig. 4d ) and quantification of western blots ( Fig. 4e ). A similar increase in total FN levels was observed after immunoblotting total cell lysates or imaging FN at the ventral surface of cells by TIRF microscopy ( Supplementary Fig. 4c,d ), further supporting the conclusion that acetylation of microtubules increases FN deposition. Interestingly, cells that had higher total levels of FN appeared to have more disorganized FN fibrils ( Fig. 4d ). Inhibition of HDAC6 has been implicated in adhesion dynamics [32] , [33] . Thus, to examine the behaviour of adhesions in cells expressing different tubulins, HFFs were co-transfected with mApple-tagged paxillin, and the leading edges of these cells were visualized over time. HFFs expressing HyperAcMT had a decreased rate of adhesion disassembly ( Fig. 4f,g ; Supplementary Movie 1 ), but unchanged assembly rate compared with the cells expressing K40A HypoAcMT ( Supplementary Fig. 4e ). Also, HFFs expressing HyperAcMT often had the elongated paxillin-containing adhesions at the front as well as the rear of the cells ( Fig. 4a,f ). Altogether, these data suggest that an increase in microtubule acetylation inhibits adhesion disassembly at the leading edge of migrating cells and increases the number of fibrillar adhesions. Microtubule acetylation alters α 5 β 1 integrin trafficking Maturation into fibrillar adhesions and FN matrix assembly require actomyosin contraction [9] , [11] , [35] . Therefore, it was surprising to find that increased acetylation of microtubules, which decreases cellular contractility ( Fig. 1 ), induced more fibrillar adhesions and FN matrix. Nonetheless, it has also been established that receptor density can influence migration rate [37] , and thus potentially influence the types and/or the strength of adhesions of cells. Expression of HyperAcMT increased surface localization of α 5 β 1 integrin compared with the cells expressing K40A HypoAcMT ( Fig. 5a,b ). We found that treatment with TSA or expression of HyperAcMT decreased internalization of α 5 β 1 , yet increased recycling of the same integrin from the recycling endosomes back to the plasma membrane ( Fig. 5c,d ). We did not see any significant change in α v β 3 integrin trafficking ( Supplementary Fig. 5 ), suggesting that the changes in acetylation of microtubules selectively affect the α 5 β 1 integrin. Taken together, these data support our initial finding that there is an increase in the surface density of α 5 β 1 integrins when acetylation of microtubules is increased. 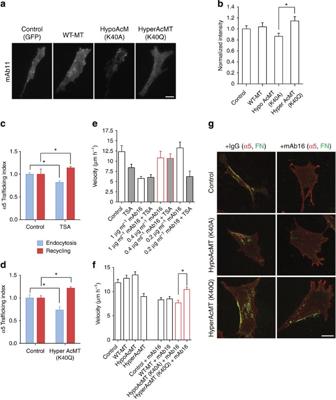Figure 5: Acetylation of microtubules increases surface density of α5β1 integrin and inhibits cell migration. (a) Representative TIRF images of HFFs expressing different tubulin mutants and immunostained with an mAb11 anti-α5 antibody without permeabilizing cell membranes. (b) Quantification ofa; intensities were normalized to the control. A minimum of 30 cells were analysed per condition (n=4). (c) Normalized level of endocytosis or recycling from recycling endosomes of α5β1 integrin after TSA treatment (n>3). (d) Normalized level of endocytosis or recycling from recycling endosomes of α5β1 integrins in cells expressing GFP (control) or GFP-tagged acetyl-mimetic tubulin (HyperAcMT) (n>4). (e) Migration velocity of HFFs treated with TSA and function-blocking antibody to α5β1 integrin (mAb16). The concentration of mAb16 reversing the TSA-induced migration defect is highlighted in red. A minimum of 40 time points were used per measurement from >10 cells per condition (n=3). (f) Migration velocity of HFFs stably expressing the indicated tubulins in the absence or presence of function-blocking antibody to α5β1 integrin (mAb16). A minimum of 40 time points were used per measurement from >29 cells per condition (n>4). (g) Representative confocal images of HFFs expressing the indicated tubulin in the presence or absence of function-blocking mAb16. FN was visualized with an anti-FN antibody (green) and α5β1 integrin with anti-α5 antibody (red). Data shown as mean±s.e.m. *P<0.05. Two-way analysis of variance (ANOVA) followed by Tukeypost testwas used forbandf, and Student’st-test was used forcandd. Scale bar, 20 μm. Figure 5: Acetylation of microtubules increases surface density of α5β1 integrin and inhibits cell migration. ( a ) Representative TIRF images of HFFs expressing different tubulin mutants and immunostained with an mAb11 anti-α5 antibody without permeabilizing cell membranes. ( b ) Quantification of a ; intensities were normalized to the control. A minimum of 30 cells were analysed per condition ( n =4). ( c ) Normalized level of endocytosis or recycling from recycling endosomes of α5β1 integrin after TSA treatment ( n >3). ( d ) Normalized level of endocytosis or recycling from recycling endosomes of α5β1 integrins in cells expressing GFP (control) or GFP-tagged acetyl-mimetic tubulin (HyperAcMT) ( n >4). ( e ) Migration velocity of HFFs treated with TSA and function-blocking antibody to α5β1 integrin (mAb16). The concentration of mAb16 reversing the TSA-induced migration defect is highlighted in red. A minimum of 40 time points were used per measurement from >10 cells per condition ( n =3). ( f ) Migration velocity of HFFs stably expressing the indicated tubulins in the absence or presence of function-blocking antibody to α5β1 integrin (mAb16). A minimum of 40 time points were used per measurement from >29 cells per condition ( n >4). ( g ) Representative confocal images of HFFs expressing the indicated tubulin in the presence or absence of function-blocking mAb16. FN was visualized with an anti-FN antibody (green) and α5β1 integrin with anti-α5 antibody (red). Data shown as mean±s.e.m. * P <0.05. Two-way analysis of variance (ANOVA) followed by Tukey post test was used for b and f , and Student’s t -test was used for c and d . Scale bar, 20 μm. Full size image To test whether the increased surface density of α 5 β 1 integrin contributes to the decreased migration rate of HFFs when microtubules are acetylated, we analysed the velocity of fibroblasts expressing HyperAcMT in the presence of low levels of function-blocking anti-α 5 β 1 antibodies [38] . Incubation with low concentrations of an inhibitory anti-α 5 β 1 antibody (0.4 μg ml −1 mAb16) rescued the fibroblast migration defect caused by the TSA treatment ( Fig. 5e ). A similar rescue was observed when cells that were transfected with HyperAcMT were incubated with the same antibody at a similar concentration ( Fig. 5f ). Moreover, this partial inhibition of α 5 β 1 integrin decreased the number of fibrillar adhesions staining positively for FN and α 5 β 1 integrin ( Fig. 5g ), suggesting that the reduced migration rate was due to changes in the surface density of α 5 β 1 integrins: that is, partial inhibition of α 5 β 1 integrin with a decrease in the number of fibrillar adhesions was sufficient to restore the migration rate to normal. Branching morphogenesis reproduces results from cell culture To verify whether the interplay between contractility and microtubule acetylation also exists in vivo , we analysed branching morphogenesis of submandibular glands (SMGs) from mice at embryonic days 12.5–13. The SMG serves as an excellent model system because it is an integrated, complex system requiring both mesenchymal–epithelial and cell–matrix interaction, and it continues to develop normally after explantation with a characteristic programme of morphogenesis to form a highly branched organ structure. Furthermore, these ex vivo cultures of SMG can be genetically and pharmacologically manipulated to study morphogenesis in detail [39] . We first immunostained SMGs to compare the physiological localization of myosin II, which correlates with local contractility [40] , and acetylated microtubules. Myosin IIA localized to the basal side of the epithelium, but acetylated microtubules localized to the apical side of the epithelial cells, the exact opposite of myosin IIA ( Fig. 6a ). A similar non-overlapping localization of myosin IIA and acetylated microtubules was observed in HFFs ( Supplementary Fig. 6a ). Moreover, treatment of SMG with TSA caused outer bud relaxation, partial flattening of the glands and fewer buds, indicating inhibition of branching morphogenesis ( Fig. 6b ). Although it is not clear which specific cells are causing these changes, these morphological changes were similar to the effects caused by low doses of blebbistatin ( Supplementary Fig. 6b ), suggesting that the interplay between actomyosin contraction and microtubule acetylation was phenocopied in intact SMG explants. Notably, similar to the findings in fibroblasts, TSA-induced hyperacetylation of microtubules in SMG increased α 5 β 1 integrin ( Fig. 6c ) and FN staining ( Fig. 6d ) at the junction between epithelium and mesenchyme. In addition, the TSA-treated glands lost the distinctive localization of myosin IIA and acetylated microtubules ( Supplementary Fig. 6c ). 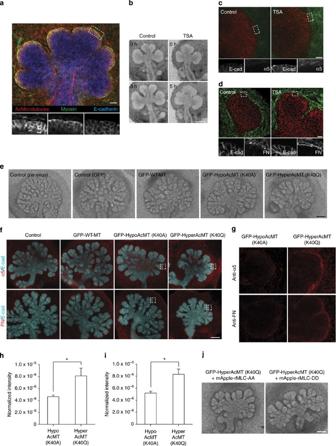Figure 6: Submandibular gland (SMG) explants also reciprocally regulate contractility and microtubule acetylation. (a) Confocal image of E13 mouse SMG explant grown on a filter membrane and immunostained for acetylated microtubules (red), myosin IIA (green) or E-cadherin (blue). In the bottom row, a representative area (hatched box) depicting the junction between the epithelium and mesenchyme is shown. (b) Representative brightfield images of paired mouse SMG explants at E13 treated with 20 μM TSA. (c,d) Representative confocal images of paired mouse SMG explants grown on a filter membrane and treated with 20 μM TSA and immunostained for α5integrin (c, green) or FN (d, green) with E-cadherin (red). In the bottom row, a representative area (hatched box) depicting the epithelium–mesenchyme junction is shown. (e) Representative brightfield images of mouse SMG explants infected with lentiviruses encoding the indicated proteins. Paired SMGs infected with GFP or GFP-WT-MT, and GFP-K40A-HypoAcMT or GFP-HyperAcMT. (f) Maximally projected confocal images of SMG explants expressing indicated proteins and immunostained for E-cadherin (teal), α5β1 integrins (red, top panels) or FN (red, bottom panels). (g) Hatched boxes infshown enlarged. Intensity of FN (h) or α5 integrin (i) normalized to intensity of E-cadherin and area of the epithelium in pixels (>8 glands;n=3). (j) Representative brightfield images of SMG explants coinfected with GFP-tagged HyperAcMT and mApple-tagged phospho-null MLC (rMLC-AA, negative) or mApple-tagged phospho-mimetic MLC (rMLC-DD, activated). Data are mean±s.e.m. *P<0.05. Scale bar, 200 μm (e,f); scale bar, 100 μm (a,b,j); and scale bar, 50 μm (c,d). Student’st-test was used forhandi. Figure 6: Submandibular gland (SMG) explants also reciprocally regulate contractility and microtubule acetylation. ( a ) Confocal image of E13 mouse SMG explant grown on a filter membrane and immunostained for acetylated microtubules (red), myosin IIA (green) or E-cadherin (blue). In the bottom row, a representative area (hatched box) depicting the junction between the epithelium and mesenchyme is shown. ( b ) Representative brightfield images of paired mouse SMG explants at E13 treated with 20 μM TSA. ( c , d ) Representative confocal images of paired mouse SMG explants grown on a filter membrane and treated with 20 μM TSA and immunostained for α 5 integrin ( c , green) or FN ( d , green) with E-cadherin (red). In the bottom row, a representative area (hatched box) depicting the epithelium–mesenchyme junction is shown. ( e ) Representative brightfield images of mouse SMG explants infected with lentiviruses encoding the indicated proteins. Paired SMGs infected with GFP or GFP-WT-MT, and GFP-K40A-HypoAcMT or GFP-HyperAcMT. ( f ) Maximally projected confocal images of SMG explants expressing indicated proteins and immunostained for E-cadherin (teal), α5β1 integrins (red, top panels) or FN (red, bottom panels). ( g ) Hatched boxes in f shown enlarged. Intensity of FN ( h ) or α5 integrin ( i ) normalized to intensity of E-cadherin and area of the epithelium in pixels (>8 glands; n =3). ( j ) Representative brightfield images of SMG explants coinfected with GFP-tagged HyperAcMT and mApple-tagged phospho-null MLC (rMLC-AA, negative) or mApple-tagged phospho-mimetic MLC (rMLC-DD, activated). Data are mean±s.e.m. * P <0.05. Scale bar, 200 μm ( e , f ); scale bar, 100 μm ( a , b , j ); and scale bar, 50 μm ( c , d ). Student’s t -test was used for h and i . Full size image To verify that the observed morphological changes and the α 5 β 1 integrin and FN staining on SMG after TSA treatment were due to increased acetylation of microtubules, different tubulin mutants were expressed in SMGs. Lentivirus-mediated expression of these exogenous proteins was extremely low, yet this barely detectable level was effective in mediating characteristic cytoskeletal modifications with no effects on viability of the cultured organs ( Supplementary Fig. 6d ). Expression of HyperAcMT in SMGs recapitulated the morphological changes seen with TSA ( Fig. 6e ): the outer bud relaxed and branching morphogenesis was inhibited even at later developmental stages (E12.5+3 days). Furthermore, similar to TSA treatment, expression of HyperAcMT increased FN and α 5 β 1 integrin at the interface between epithelial and mesenchymal cells ( Fig. 6f–i ), indicating that the changes observed in cultured fibroblasts on this integrin and FN are recapitulated in intact SMG. Our findings from fibroblast studies also predicted that counterbalancing the increased microtubule acetylation with a concomitant increase in contractility should rescue the morphological defect observed in SMG. As predicted, coexpression of rMLC-DD rescued the morphological defect while rMLC-AA did not ( Fig. 6j ). As noted above, lentiviral expression of GFP- or mApple-tagged proteins was extremely low, minimizing concerns about overexpression artefacts ( Supplementary Fig. 6e ). These findings provide evidence that microtubule acetylation plays a role in branching morphogenesis and, consistent with our findings in cultured cells, evidence that the interplay between cellular contractility and microtubule acetylation is also important in an intact organ containing both epithelium and mesenchyme. Interestingly, expression of rMLC-DD alone severely hindered branching morphogenesis ( Supplementary Fig. 6f ), indicating the importance of an appropriate balance in this organ system. Altogether, these data indicate that findings in cultured fibroblasts are recapitulated in an in vivo model system of development. Many groups have reported cross-talk between the actin cytoskeleton and microtubule networks. However, these documented systems of cross-talk describe how the polymerization and depolymerization of the two cytoskeletal systems are coordinated by controlling the availability of signalling components such as Rac1 and RhoA GTPases, their regulators, such as GEFs, GAPs, or other downstream effectors or by regulating the molecular scaffolding platform for the two cytoskeletons [15] , [41] , [42] , [43] , [44] , [45] , [46] , [47] , [48] . The biological effects described in this paper were independent of effects on microtubule dynamics. Our data provide the first evidence demonstrating cross-talk between actin cytoskeleton and microtubule networks post-polymerization in which cellular contractility is inversely regulated by microtubule acetylation; the mechanism is through interaction with myosin phosphatase. Our working model ( Fig. 7 ) suggests that actomyosin-mediated cellular contractility and acetylation of microtubules are also spatially coordinated, since activation of myosin phosphatase would decrease local actomyosin contraction but increase microtubule acetylation. As predicted by this model, acetylated microtubules and myosin II localization, used previously as an indicator of contractility [40] , do not co-localize in fibroblasts and SMGs. In fact, there seems to be exclusive and generally non-overlapping localization of the two types of cytoskeletons. We speculate that this spatial coordination reflects a competitive sequestration process where changes in acetylation of microtubules trap HDAC6–myosin phosphatase complex to microtubules thereby decreasing the amount of free MYPT1 available to interact with MLC, or a sequestration of HDAC6 by transfected acetyl-mimetic tubulins that result in a modification of HDAC6 activity elsewhere in the cell. 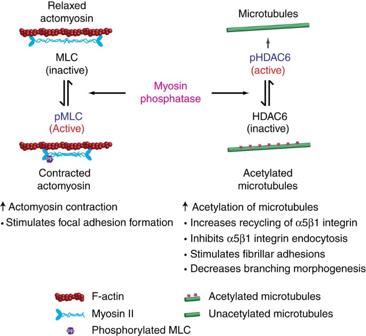Figure 7: Schematic summary of the role of MYPT1 in regulating contractility and microtubule acetylation. A model for MYPT1 as a molecular switch that reciprocally modulates the level of actomyosin-mediated cellular contractility and microtubule acetylation. When MYPT1 binds and dephosphorylates MLC or HDAC6, cellular contractility is decreased or HDAC6 activity is inhibited with increased acetylation of microtubules, respectively. Conversely, when MYPT1 is not bound to MLC, cellular contractility is enhanced due to increased phosphorylation of MLC; when not bound to MYPT1, HDAC6 activity is increased and promotes deacetylation of microtubules. Figure 7: Schematic summary of the role of MYPT1 in regulating contractility and microtubule acetylation. A model for MYPT1 as a molecular switch that reciprocally modulates the level of actomyosin-mediated cellular contractility and microtubule acetylation. When MYPT1 binds and dephosphorylates MLC or HDAC6, cellular contractility is decreased or HDAC6 activity is inhibited with increased acetylation of microtubules, respectively. Conversely, when MYPT1 is not bound to MLC, cellular contractility is enhanced due to increased phosphorylation of MLC; when not bound to MYPT1, HDAC6 activity is increased and promotes deacetylation of microtubules. Full size image It is surprising that blebbistatin treatment increases pMLC levels when the reagent directly inhibits ATPase function of myosin II [49] . However, others have observed similar increases in pMLC upon blebbistatin treatment [21] . A possible explanation is that HFFs treated with blebbistatin may make a futile attempt to compensate for a lack of contractility by increasing pMLC levels. Mechanistically, treatment with blebbistatin decreased the quantity of HDAC6–MYPT1 complex, similar to TSA treatment, which would account for the increased acetylation of microtubules after blebbistatin treatment. We were intrigued by our finding that branching morphogenesis was inhibited after disruption of the balance between contractility and microtubule acetylation. Furthermore, similar to our single-cell migration studies, the defect in branching morphogenesis due to hyperacetylation of microtubules was partially rescued by experimentally increasing contractility. These results suggest that altered contractility disrupts the myosin II-dependent processes critical for organ branching [50] , that decreased contractility due to hyperacetylation fails to support the local tension needed for basement membrane remodelling during morphogenesis [51] , and/or that the accompanying increases in α 5 β 1 integrin and FN at the junction between epithelium and mesenchyme hinder the epithelial cell motility associated with the tissue remodelling of branching morphogenesis [52] , [53] . We speculate that a combination of these factors is responsible for the inhibition of epithelial branching morphogenesis after altering the balance of microtubule acetylation and contractility. In summary, we have identified a new molecular mechanism involving MYPT1 for achieving post-polymerization cross-talk between the actin cytoskeleton and microtubule networks. Furthermore, this novel cross-talk appears to be needed for optimal density of α 5 β 1 integrin, attachment to the substrate and FN matrix organization, thus helping to regulate migration rate and epithelial branching morphogenesis. Plasmids and reagents pEGFPN1-MLC and pEGFPN1-MLC (18D19D) were gifts from K. Kelly (NIH), and pmApple-paxillin was a gift from M. Davidson (Florida State University). pEGFP-Tub, Flag-HDAC6 (Addgene plasmid 13,823) [54] , pk.myc-MYPT1 (Addgene plasmid 24,101) [55] , pRSV-Rev (Addgene plasmid 12,253) [56] , pCMV-VSV-G (Addgene plasmid 8,454) [57] , pLL3.7 (Addgene plasmid 11,795) [58] and pMDLg/pRRE (Addgene plasmid 12,251) [56] were obtained from Clontech or Addgene. All mutageneses were carried out using Quick Change Lightening Site-Directed mutagenesis kit (Stratagene) using the following templates: pEGFPN1-MLC served as a template to make pEGFPN1-MLC (18A19A) using forward PCR primer 5′-(CGCAGCGCGCCGCCGCCAATGTCTTCGC)-3′ and reverse PCR primer 5′-(GCGAAGACATTGGCGGCGGCGCGCTGCG)-3′; pEGFP-Tub served as a template to make pEGFP-α-tubulin-K40A (acetyl-null) using forward PCR primer 5′-(CCAGATGCCAAGTGACGCGACCATTGGGGGAGGA)-3′ and reverse PCR primer 5′-(TCCTCCCCCAATGGTCGCGTCACTTGGCATCTGG)-3′; pEGFP-α-tubulin-K40R (acetyl-null) using forward PCR primer 5′-(AGATGCCAAGTGACAGGACCATTGGGGGGAGG)-3′ and reverse PCR primer 5′-(CCTCCCCCAATGGTCCTGTCACTTGGCATCT)-3′; and pEGFP-α-tubulin-K40Q (acetyl-mimetic) using forward PCR primer 5′-(CAGATGCCAAGTGACCAGACCATTGGGGGAG)-3′ and reverse PCR primer 5′-(CTCCCCCAATGGTCTGGTCACTTGGCATCTG)-3′; Flag-HDAC6 served as a template to make Flag-S22A-HDAC6 using forward PCR primer 5′-(CAGAACCCCCAGGCGCCCCCTCAGG)-3′ and reverse PCR primer 5′-(CCTGAGGGGGCGCCTGGGGGTTCTG)-3′; or Flag-S22E-HDAC6 using forward PCR primer 5′-(GCAGAACCCCCAGGAGCCCCCTCAGGAC)-3′ and reverse PCR primer 5′-(GTCCTGAGGGGGCTCCTGGGGGTTCTGC)-3′. pGEX4T-MYPT1 was made by subcloning MYPT1 into pGEX4T (GE Healthcare), pET28-HDAC6 by subcloning HDAC6 into pET28 (Novagen), pLL3.7-Tub by subcloning pEGFP-Tub into pLL3.7, pLL3.7-α-tubulin-K40A by subcloning pEGFP-α-tubulin-K40A into pLL3.7 and pLL3.7-α-tubulin-K40Q by subcloning pEGFP-α-tubulin-K40Q into pLL3.7. To make pLL3.7-mApple-MLC (18A19A), pmApple-MLC (18A19A) was first made by subcloning pEGFPN1-MLC (18A19A) into pmApple-paxillin, to replace paxillin with MLC (18A19A), then subcloning pmApple-MLC (18A19A) into pLL3.7. pLL3.7-mApple-MLC (18D19D) was made in a similar manner as pLL3.7-MLC (18A19A). pmApple-tagged EB1 was made by subcloning pGFP-EB1 (Addgene plasmid 17,234) [59] into pmApple-paxillin between NheI and SmaI restriction sites to replace paxillin with EB1. TSA and calyculin A were from Sigma, and blebbistatin and ML-7 were from Calbiochem. Microdishes of 28 kPa were from ibidi, and rat tail collagen was from BD Biosciences. An anti-acetylated tubulin antibody (Sigma, T6793) was used at 1:2,000 dilution for western blots or 1:500 for immunostaining, an anti-GAPDH antibody (Fitzerald, 10R-G109a) was used at 1:10,000 dilution for western blots, an anti-pMLC antibody (Abcam, ab2480) was used at 1:5,000 dilution for western blots, an anti-MYPT1 antibody (BD Biosciences, 612,165) was used at 1:1,750 dilution for western blots, an anti-HDAC6 antibody (Millipore, 07-732) was used at 1:1,000 dilution for western blots, an anti-MLC (Rockland, 600-491-938) was used for immunoprecipitation, an anti-pSer antibody (Cell Signaling, 2,325) was used at 1:1,000 dilution for western blots, an anti-Flag antibody (Thermo Scientific, MA1-91878) was used at 1:1,000 dilution for western blots, an anti-fibronectin antibody (clone #5836 or clone #3B8) was used at 1:1,000 dilution for western blots or 1:200 for immunostaining, an anti-Paxillin antibody (BD Bioscience, 610,619) was used at 1:100 for immunostaining, an mAb11 was used at 1:200 for immunostaining, an mAb16 was used at 1:200 for immunostaining, an anti-α5 integrin antibody (BD Bioscience, 555,650 or 553,319) was used at 1:200 dilution, an anti-Myosin IIA (Covance, PRB-440P) was used at 1:200 for immunostaining, an anti-E-cadherin antibody (Invitrogen, 13-1900) was used at 1:200 for immunostaining, an anti-β3 integrin (BD Biosciences, 555,752) was used at 1:200 for immunostaining and an anti-pTyr antibody (Millipore, 05-1050) was used at 1:200 for immunostaining. siRNA duplexes targeting MYPT1 5′-(CAACUAAACAGGCCAAAUA-3′, 5′-GCUAAAUAGUGGUCAUAUA, 5′-ACAAAGAGACGUUGAUUAU-3′, 5′-CGGAUUCCAUUUCUAGAUA), HDAC6 5′-(GGGAGGUUCUUGUGAGAUC-3′, 5′-GGAGGGUCCUUAUCGUAGA-3′, 5′-GCAGUUAAAUGAAUUCCAU-3′, 5′-GUUCACAGCCUAGAAUAUA)-3′ or control 5′-(UGGUUUACAUGUCGACUAA-3′, 5′-UGGUUUACAUGUUGUGUGA-3′, 5′-UGGUUUACAUGUUUUCUGA-3′, 5′-UGGUUUACAUGUUUUCCUA)-3′ were from Dharmacon. Cell culture and lysates HFFs were gifts from M. dos Santos and were cultured as described [18] . Cell lysates from HFF were obtained by plating 1.2 × 10 5 cells per 35 mm dish and treating them the following day with 5 μM TSA, 25 μM blebbistatin, 20 μM ML-7 for 1 h at 37 °C or with 10 nM calyculin A for 20 min before lysing with RIPA buffer (50 mM Tris 7.5, 150 mM NaCl, 1% NP-40, 0.5% sodium deoxycholate, 0.1% SDS) supplemented with 2 × protease inhibitors (Roche) and 2 × phosphatase inhibitors (Roche). In addition, cell lysates from HFF were obtained after transfecting 50–100 nM pooled siRNA towards HDAC6, MYPT1 or scrambled control (Thermo Fisher Scientific) with Lipofectamine 2,000 (Invitrogen) for 72 h then lysing with RIPA buffer. Finally, HFF cell lysates were obtained after eletroporating S22A-HDAC6, S22E-HDAC6 or wild-type HDAC6 plasmids with Amaxa transfection reagent (Lonza) then lysing with RIPA buffer. For clarity, western blots were cropped to show the band of interest in the main figures. However, each corresponding uncropped western blot can be found in Supplementary Fig. 7 . Local collagen contraction assay A total of 2 × 10 4 HFF cells per ml were mixed with 1.8 mg ml −1 rat tail collagen (BD Biosciences) and plated on a glass-bottom dish (MatTek) containing a thin layer of prepolymerized rat tail collagen at 1.8 mg ml −1 and were grown overnight. Cells were then treated with drugs, if applicable, fixed with 4% paraformaldehyde and stained for actin filaments with labelled phalloidin (1:200; Invitrogen). Intensity of collagen fibres was obtained by confocal reflection by first determining the area of each cell by phalloidin staining using average threshold in MetaMorph software (Molecular Devices) followed by quantifying the average intensity of collagen fibres from the measured area. Differences of intensity of collagen fibres were then compared with the control. To ensure that the optimum distance from the coverslip was maintained between samples, all imaging was done on the same day at a similar Z distance from the coverslips. Traction force assay Traction force was measured as previously described [60] , [61] . In brief, HFFs stably expressing pEGFP-Tub, pEGFP-α-tubulin-K40A, pEGFP-α-tubulin-K40R and pEGFP-α-tubulin-K40Q were seeded on polyacrylamide (PAA) gels containing 200 nm fluorescent microspheres (Invitrogen). These polyacrylamide gels had a rigidity of 34,263 Pa, and soluble FN was coupled to them covalently. Movements of the microspheres were recorded and quantified as previously described [61] , [62] with a regularization parameter of 1.0 × 10 −9 . Immunocytochemistry and microscopy Cultured cells were first fixed to visualize adhesions [35] or by a two-step fixation to visualize microtubules and actin cytoskeleton [63] , then immunostained for different cellular components as described [64] . Anti-paxillin and anti-α5 integrin antibodies were from BD Biosciences. Confocal microscopy images were obtained using the confocal microscope and specific settings described [65] or by use of an LSM710 confocal microscope (Carl Zeiss) equipped with similar settings. Time-lapse images of mApple-paxillin-positive adhesions were acquired every 3 s for 30–60 min using a spinning disc confocal microscope as described [66] . Time-lapse images of whole cells were recorded every 5 min for 12–24 h on an inverted microscope (Axiovert 100; Carl Zeiss) using plan-Neofluar 5 × 0.16 NA or plan-Neofluar 10 × 0.3 NA phase contrast objectives (Carl Zeiss). Immunoprecipitation and protein–protein interaction Immunoprecipitation was performed as described [64] using Protein A/G Dynabeads (Invitrogen) and probed for MYPT1 (1:1,750, BD Biosciences), HDAC6 (1:1,000, Millipore) or pSer (1:1,000, Cell Signaling). Immunoprecipitation for HDAC6 that was to probe with a pSer antibody was done using RIPA buffer supplemented with 300 mM NaCl. Full-length recombinant HDAC6 was generated in BL21 cells and purified using the T7 tag affinity purification system (Millipore). Full-length GST-tagged recombinant MYPT1 was purified as described [67] . Direct binding of HDAC6 and MYPT1 was assayed by incubating equal molar concentrations of immobilized GST-tagged MYPT1 with eluted T7-tagged HDAC6 in PBS supplemented with 1 mM DTT and protease and phosphatase inhibitors (Roche) for 12–16 h at 4 °C. For competition assays, purified HDAC6 protein (<100 μg) was added to the whole-cell lysate before immunoprecipitation. Integrin trafficking and adhesion dynamics Endocytosis and recycling measurement were performed as described [68] . Fluorescence intensity of mApple-paxillin positive adhesions at the leading edge was plotted over time, and ascending (assembly rate) and descending slopes (disassembly rate) were measured [10] . Cell migration For measuring migration velocities, the nuclei of migrating cells were tracked using MetaMorph software, and instantaneous velocity was measured for 30–60 time points. When necessary, TSA and the function-blocking antibody were incubated at the same time. Microtubule dynamics and immunostaining HFFs stably expressing pEGFP, pEGFP-Tub, pEGFP-α-tubulin-K40A or pEGFP-α-tubulin-K40Q were electroporated with pmApple-tagged EB1 using the NHDF Nucleofector Kit (Lonza) following the manufacturer’s instructions. Movements of mApple-tagged EB1 were measured, and growth, shortening and pause were quantified as previously described [69] . Cultured cells were fixed as previously described [63] . In brief, cells were first incubated in 1 mM dithiobis (succinimidylpropionate) crosslinker (DSP; Pierce) in Hanks’ balanced salt solution (Life Technologies) for 10 min, followed by 1 mM DSP in TSB buffer (0.5% Triton X-100, 1 mM EGTA, 4% polyethylene glycol 8,000, 100 mM PIPES, pH 6.9) for 10 min. Cells were washed with TSB buffer for 5 min and fixed with 4% paraformaldehyde (Electron Microscopy Sciences) in MTSB buffer (1 mM EGTA, 4% polyethylene glycol 8,000, 100 mM PIPES, pH 6.9) for 15 min. The cells were then immunostained with anti-tubulin (1:500; Sigma) or anti-acetylated tubulin (1:500; Sigma) antibodies. Submandibular gland studies All animal maintenance and procedures were in accordance with guidelines of the Intramural Program of the National Institutes of Health under National Institute of Dental and Craniofacial Research Animal Care and Use Committee protocol number 11–634. SMGs were dissected from ICR mice at embryonic day 12.5–13.5 (ref. 70 ), cultured on either 0.1 or 0.2 μm polycarbonate membrane filters (Whatman), and grown at 37 °C, 5% CO 2 in DMEM/F12 media supplemented with 1% transferrin (Sigma) and 0.2% ascorbic acid (Sigma). To assay the effect of TSA, SMGs were cultured overnight on 0.1 μm filters and treated with 20 μM TSA for up to 5 h, and images were acquired using an inverted brightfield microscope. SMGs were immunostained as described [70] . In brief, organ cultures were first fixed with either 4% paraformaldehyde for 15 min, then permeabilized with 0.5% Triton X-100/100 mM glycine at room temperature for 5–10 min or fixed with a methanol:acetone (1:1) mixture at −20 °C for 15 min with no further permeabilization. Glands were then incubated with blocking buffer (0.05% Tween-20, 5% donkey serum, 1% BSA and MOM blocking reagent (Vector Laboratories) in PBS) before incubating with either primary or secondary antibodies in PBS supplemented with 0.05% Tween-20, 5% donkey serum and 8% MOM protein (Vector Laboratories) at 4 °C overnight. Antibody incubation was followed by extensive washes with PBS supplemented with 0.05% Tween-20. Immunostained glands were imaged from the top to the bottom of the epithelium at optimal, equal z -distances for each set of experiments (1.7–2.7 μm). To quantify FN staining intensity, z -sectioned images were collapsed using the maximum projection function using Zen software (Carl Zeiss), and intensity was measured using MetaMorph software and then normalized against E-cadherin staining and area. For exogenous expression of different tubulins at low amounts in cultured salivary glands, lentivirus was generated as described [58] and concentrated using PEG-it solution (System Biosciences). A total of 2 × 10 8 virus titre was used to infect each set of glands for 2–3 days. Glands were allowed to recover from the virus infection for 18–24 h before fixing as described above. Statistical analysis Sample sizes for each statistical analysis were based on current literature standards. For analyses of single-cell migration, cells undergoing mitosis were excluded from analyses. Comparisons between two groups were analysed by the Student’s t -test, while multiple group comparisons were first analysed by two-way analysis of variance (ANOVA) followed by Tukey post test . Differences were considered significant at P <0.05 with n indicating the number of independent experiments. How to cite this article: Joo, E. E. et al. MYPT1 regulates contractility and microtubule acetylation to modulate integrin adhesions and matrix assembly. Nat. Commun. 5:3510 doi: 10.1038/ncomms4510 (2014).